Cdkn1b overexpression in adult mice alters the balance between genome and tissue ageing Insufficient cell proliferation has been suggested as a potential cause of age-related tissue dysgenesis in mammals. However, genetic manipulation of cell cycle regulators in the germ lines of mice results in changes in animal size but not progeroid phenotypes. Here we increase levels of the cyclin-dependent kinase inhibitor Cdkn1b (p27kip1) in adult mice through doxycycline-inducible expression and show this results in reduced cell proliferation in multiple tissues. The mice undergo changes resembling ageing even in the absence of an elevated DNA damage response or evidence of senescent cells, suggesting an altered balance between genetic and tissue ageing. In contrast, suppressing cell proliferation by doxycycline treatment of neonates retards growth, but the onset of degenerative changes is delayed during the period of reduced body mass. These results support the hypothesis that many of the most recognizable features of mammalian ageing can result from an imbalance between cell production and the mass of tissue that must be maintained. Accumulation of genetic damage in somatic tissue has been postulated to contribute to mammalian ageing [1] , [2] . Further, progeroid phenotypes are observed when mechanisms that maintain genome integrity (for example, telomerase [3] , Ercc1 (ref. 4 ) and BubR1 (ref. 5 )) are compromised. Additional studies suggest that effects of genetic damage are indirect, resulting from induction of DNA damage response pathways. On DNA damage, p53 and/or Rb signalling pathways are induced, leading to elevation of the cyclin-dependent kinase inhibitors Cdkn1a (p21) and/or Cdkn2a (p16 Ink4a ), and either temporary or permanent cell cycle arrest [6] . One explanation for the progeroid phenotypes of mutations affecting genome integrity is that cell proliferation is suppressed to a level that causes tissue dysfunction [7] . In support of this idea, senescent cells accumulate in mammalian tissues with age, and both Cdkn1a and Cdkn2a are elevated in their expression [8] . Further, deletion of Cdkn1a or Cdkn2a has been shown to rescue progeroid phenotypes resulting from mutations that compromise genome integrity. For example, germline deletion of Cdkn1a delays the progeroid phenotype that occurs in late-generation telomerase knockout mice [9] . Similarly, germline deletion of Cdkn2a delays the premature ageing of BubR1 mutant mice [10] . In the context of otherwise normal mice, Cdkn2a deletion has been shown to result in a partial rescue of the decrease in stem/progenitor cell survival or function that occurs during ageing in at least a subset of tissues [11] , [12] , [13] and germline deletion of Cdkn1a has been shown to increase stem and progenitor cell proliferation in a variety of specific tissues in vivo [14] , [15] , [16] . However, in the subventricular zone (SVZ) of the brain [14] and haematopoietic system [16] , an early elevation in proliferation of neural stem cells (NSCs) or hematopoietic stem cells (HSCs) in Cdkn1a knockout mice is followed by reduced stem cell numbers later in life, consistent with stem cell exhaustion. The phenotypes resulting when levels of an additional cyclin-dependent kinase, Cdkn1b (p27), are modulated are also relevant to the consequences of modulating cell proliferation for tissue maintenance. Cdkn1b is not directly induced by p53 or Rb, and does not show elevated expression during ageing. Instead, it is regulated by extracellular antiproliferative signals, including contact inhibition or serum deprivation [17] , [18] . Nonetheless, transgenic models in which the levels of Cdkn1b are affected do exhibit altered cell proliferation in the in vivo situation. Cdkn1b-null mice grow to approximately twice the normal size and exhibit organomegaly [19] , [20] . They develop pituitary adenomas by 10 weeks of age with high penetrance; hence, the effect on overall longevity is not known. Conversely, it has been possible to determine the effect of elevated Cdkn1b expression, as Cdkn1b is a primary target of the Culin-RING ubiquitin ligase SCF Skp2 , which mediates its degradation. Skp2-null mice exhibit elevated levels of Cdkn1b, reduced proliferation in many tissues and grow to <75% of the size of wild-type (wt) animals [21] . Nonetheless, Skp2-null mice do not exhibit premature tissue degeneration. The lack of age-related phenotypes in these mice poses a particular challenge to the idea that insufficient cell proliferation accounts for age-related tissue dysfunction. Here the consequences of reduced cell proliferation in multiple tissues of adult mice are assessed through the ectopic expression of Cdkn1b (p27 kip1 ) under doxycycline-inducible control. In sharp contrast to the phenotype of germline Skp2-knockout mice, doxycycline-induced overexpression of Cdkn1b in adult animals results in many changes that are characteristic of advanced age at both the gross phenotypic and histological levels within a few months of treatment. Cdkn1b expression in Tre-Tight-Cdkn1b transgenic mice A line of transgenic mice in which Cdkn1b (p27 kip1 ) is expressed from the TreTight promoter (TreTight-Cdkn1b) was constructed and mated with ROSA26-TetON (R26-M2rtTA) transgenic mice to create R26-M2rtTA;TRE-Tight-Cdkn1b bigenic mice. Cdkn1b expression is under tight control of doxycycline in R26-M2rtTA;TRE-tight-Cdkn1b transgenic mice. 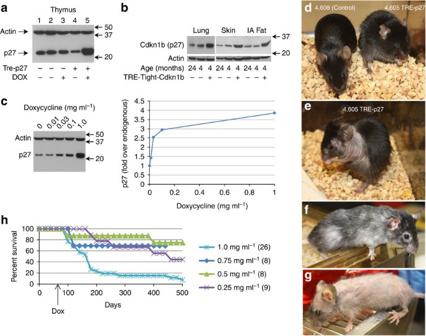Figure 1: Induction of Cdkn1b protein and phenotypic changes in R26-M2rtTA;TRE-Tight-Cdkn1b transgenic mice. (a) Western blotting showing Cdkn1b (p27) and actin in thymuses of mice carrying the R26-M2rtTA transgene with or without the TreTight-Cdkn1b transgene or treatment with 1 mg ml−1doxycycline (Dox) for 24 h (a full-length image of this blot is shown inSupplementary Fig. 10a). (b) Cdkn1b protein levels in the lung, skin and intra-abdominal fat of R26-M2rtTA transgenic mice that either carry or do not carry the TRE-Tight-Cdkn1b transgene, where, starting at 2 months of age, mice were continuously treated with 1 mg ml−1Dox for 2 months and assessed at 4 months of age. In addition, Cdkn1b expression in the same tissues from a control 24-month-old mouse is included for comparison. (c) A titration of Dox concentration versus Cdkn1b expression in the thymus of mice that were treated with the indicated concentrations of Dox for 3 days. Western blotting is shown on the left and quantified by densitometry of Cdkn1b levels corrected for loading based on the signal from actin on the right. Arrows to the right ofa–cindicate the positions of size markers in kDa. (d) Gross phenotypic changes in an R26-M2rtTA control (left, mouse 4608) and R26-M2rtTA;TreTight-Cdkn1b (right, mouse 4605) mice continuously treated with 1 mg ml−1Dox beginning at 2 months of age for a period of 3 weeks. The same R26-M2rtTA;TreTight-Cdkn1b mouse is also shown at 6 weeks (e) or 5 months (f) of continuous Dox administration. (g) A mouse treated, beginning at 2 months of age, continuously for 9 months with 0.75 mg ml−1Dox. (h) Survival in days of R26-M2rtTA;TreTight-Cdkn1b mice treated with various concentrations of Dox as indicated in the figure, where the number of mice per group is given in parentheses. None of 40 Cdkn1b-overexpressing mice that have died during Dox treatments with doses ranging from 0.25 to 1.0 mg ml−1had overt tumours on necropsy (a rate of <2.5%). This is much lower than the expected rate for this strain (40%). In the present study, one of the four control animals that died (25%) succumbed to thymic lymphoma. Figure 1a shows Cdkn1b expression levels in the thymus from R26-M2rtTA− and R26-M2rtTA+ mice, which either do or do not carry the TRE-Tight-Cdkn1b transgene and which have been treated, or are untreated, with 1 mg ml −1 doxycycline in their drinking water. Cdkn1b expression over endogenous levels is evident only in R26-M2rtTA;TRE-Tight-Cdkn1b mice that have received doxycycline. In addition, the level of ectopic Cdkn1b expression is doxycycline dosage dependent ( Fig. 1c ) and the expression remains at elevated levels during prolonged doxycycline treatment in most tissues ( Fig. 1b ). Figure 1: Induction of Cdkn1b protein and phenotypic changes in R26-M2rtTA;TRE-Tight-Cdkn1b transgenic mice. ( a ) Western blotting showing Cdkn1b (p27) and actin in thymuses of mice carrying the R26-M2rtTA transgene with or without the TreTight-Cdkn1b transgene or treatment with 1 mg ml −1 doxycycline (Dox) for 24 h (a full-length image of this blot is shown in Supplementary Fig. 10a ). ( b ) Cdkn1b protein levels in the lung, skin and intra-abdominal fat of R26-M2rtTA transgenic mice that either carry or do not carry the TRE-Tight-Cdkn1b transgene, where, starting at 2 months of age, mice were continuously treated with 1 mg ml −1 Dox for 2 months and assessed at 4 months of age. In addition, Cdkn1b expression in the same tissues from a control 24-month-old mouse is included for comparison. ( c ) A titration of Dox concentration versus Cdkn1b expression in the thymus of mice that were treated with the indicated concentrations of Dox for 3 days. Western blotting is shown on the left and quantified by densitometry of Cdkn1b levels corrected for loading based on the signal from actin on the right. Arrows to the right of a – c indicate the positions of size markers in kDa. ( d ) Gross phenotypic changes in an R26-M2rtTA control (left, mouse 4608) and R26-M2rtTA;TreTight-Cdkn1b (right, mouse 4605) mice continuously treated with 1 mg ml −1 Dox beginning at 2 months of age for a period of 3 weeks. The same R26-M2rtTA;TreTight-Cdkn1b mouse is also shown at 6 weeks ( e ) or 5 months ( f ) of continuous Dox administration. ( g ) A mouse treated, beginning at 2 months of age, continuously for 9 months with 0.75 mg ml −1 Dox. ( h ) Survival in days of R26-M2rtTA;TreTight-Cdkn1b mice treated with various concentrations of Dox as indicated in the figure, where the number of mice per group is given in parentheses. None of 40 Cdkn1b-overexpressing mice that have died during Dox treatments with doses ranging from 0.25 to 1.0 mg ml −1 had overt tumours on necropsy (a rate of <2.5%). This is much lower than the expected rate for this strain (40%). In the present study, one of the four control animals that died (25%) succumbed to thymic lymphoma. Full size image Cdkn1b overexpression in adults induces a progeroid phenotype The gross phenotypic effects of Cdkn1b overexpression are shown in Fig. 1d–g . Phenotypic changes first become apparent at ~2–3 weeks and manifest as a change in posture, ruffled fir and transient diarrhoea that resolves over a period of ~2–3 weeks ( Fig. 1d ). An obvious nuchal to caudal wave of hair loss occurs at approximately the time of the second telogen (postnatal day 45–70 (ref. 22 ), which is consistent with delayed or inefficient re-initiation of hair growth ( Fig. 1e ). Over time, hair growth is re-established to varying degrees but is typically reduced in density and exhibits loss of pigmentation ( Fig. 1f–g ). Additional macroscopic changes occur over time, including thinning skin and lesions, loss of corneal transparency and generalized frailty. The time at which phenotypic changes occur is delayed in mice treated with lower doses of doxycycline, at least through 0.25 mg ml −1 ; however, the severity of changes is similar. Survival of mice treated with varying doses of doxycycline is shown in Fig. 1h . Loss of mice during the first 4–6 weeks, particularly at the highest dose, results from gastrointestinal problems (see below). Histological examinations of several tissues were performed for Cdkn1b-overexpressing mice in comparison with controls. Abdominal skin is shown in Fig. 2a (R26-M2rtTA+ control that does not carry TRE-Tight-Cdkn1b) and Fig. 2b (R26-M2rtTA;TRE-Tight-Cdkn1b) for mice treated with 0.25 mg ml −1 doxycycline for a period of 5 months and confirms that Cdkn1b overexpression results in a reduction in skin thickness to approximately half of that of control mice. The majority of this reduction is a consequence of loss of adipose tissue from the hypodermal layer. Gastrocnemius and abdominal muscles are shown in Fig. 2c–f . In each case, the diameter of individual fibres is reduced in Cdkn1b-overexpressing mice ( Fig. 2g,h ). 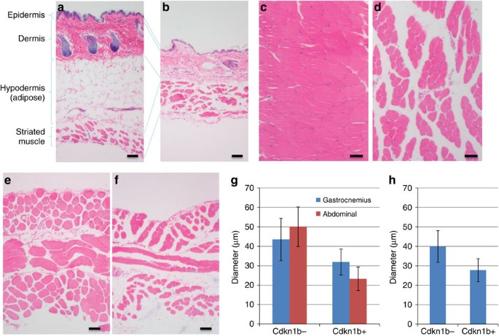Figure 2: Histological changes in skin and muscle of Cdkn1b overexpressing mice. For this set of experiments, R26-M2rtTA;TRE-Tight-Cdkn1b (b,d,f) and control (R26-M2rtTA+ littermates that do not carry the TRE-Tight-Cdkn1b transgene (a,c,e) mice were treated, beginning at 2 months of age, with 0.25 mg ml−1doxycycline (Dox) continuously for a period of 5 months. Histological sections were prepared from the abdominal skin (a,b), gastrocnemius muscle (c,d) and abdominal muscle (e,f), and stained with haematoxylin and eosin before image capture using a × 10 objective. Various layers of the skin are indicated foraandb. Ing, the diameters were determined for gastrocnemius and abdominal muscle fibres (n=50, error bars indicate s.d.) from control and R26-M2rtTA;TRE-Tight-Cdkn1b mice treated, beginning at 2 months of age, with 0.25 mg ml−1Dox continuously for a period of 5 months and show a decrease in Cdkn1b-overexpressing mice (gastrocnemiusρ=7.1 × 10−7; abdominalρ=4.8 × 10−21; two-tailed Student’st-test). (h) Muscle fibre diameters were determined for gastrocnemius muscle of control and R26-M2rtTA;TRE-Tight-Cdkn1b mice (n=50, error bars indicate s.d.) that were treated beginning at 2 months of age with 0.5 mg ml−1Dox continuously for a period of 8 months and also show a decrease in Cdkn1b-overexpressing mice (ρ=6.2 × 10−27; two-tailed Student’st-test). Scale bars ina–findicate 50 μm. Figure 2: Histological changes in skin and muscle of Cdkn1b overexpressing mice. For this set of experiments, R26-M2rtTA;TRE-Tight-Cdkn1b ( b , d , f ) and control (R26-M2rtTA+ littermates that do not carry the TRE-Tight-Cdkn1b transgene ( a , c , e ) mice were treated, beginning at 2 months of age, with 0.25 mg ml −1 doxycycline (Dox) continuously for a period of 5 months. Histological sections were prepared from the abdominal skin ( a , b ), gastrocnemius muscle ( c , d ) and abdominal muscle ( e , f ), and stained with haematoxylin and eosin before image capture using a × 10 objective. Various layers of the skin are indicated for a and b . In g , the diameters were determined for gastrocnemius and abdominal muscle fibres ( n =50, error bars indicate s.d.) from control and R26-M2rtTA;TRE-Tight-Cdkn1b mice treated, beginning at 2 months of age, with 0.25 mg ml −1 Dox continuously for a period of 5 months and show a decrease in Cdkn1b-overexpressing mice (gastrocnemius ρ =7.1 × 10 −7 ; abdominal ρ =4.8 × 10 −21 ; two-tailed Student’s t -test). ( h ) Muscle fibre diameters were determined for gastrocnemius muscle of control and R26-M2rtTA;TRE-Tight-Cdkn1b mice ( n =50, error bars indicate s.d.) that were treated beginning at 2 months of age with 0.5 mg ml −1 Dox continuously for a period of 8 months and also show a decrease in Cdkn1b-overexpressing mice ( ρ =6.2 × 10 −27 ; two-tailed Student’s t -test). Scale bars in a – f indicate 50 μm. Full size image Stem and progenitor cell cycling in Cdkn1b-overexpressing mice To measure the effect of Cdkn1b expression on cell proliferation, R26-M2rtTA;TRE-Tight-Cdkn1b transgenic mice were treated with doxycycline for various periods and administered 5-iododeoxyuridine (IdU) continuously for 3 days and 5-chlorodeoxyuridine (CldU) as a pulse 2 h before killing. Histological sections were prepared for the SVZ of the brain, a site of active neural stem cell proliferation in adults, as shown in Fig. 3a–f and Supplementary Fig. S1 . Results from this study show that within 3 days of the start of 1.0 mg ml −1 doxycycline treatment, cells incorporating nucleoside analogues are reduced to ~1/5th the level of wt mice and that this reduction in the level of division is maintained throughout at least 5 months of treatment ( Fig. 3g ). 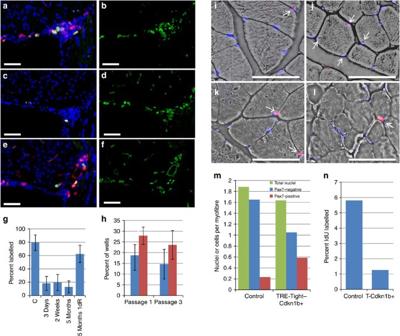Figure 3: Proliferating and replication competent cells in the brain and muscles of R26-M2rtTA;TRE-Tight-Cdkn1b mice. Supraventricular zones from R26-M2rtTA;TRE-Tight-Cdkn1b mice either untreated (a,b) or treated with 1 mg ml−1doxycycline (Dox) between months 2 and 7 (c,d) or treated between months 2 and 7 but removed from Dox treatment for 24 h (e,f). IdU was administered for 3 days (a–d) or 1 day (e,f) and CldU was administered 2 h before killing. (a,c,e) Stained for IdU (red), CldU (green) and DAPI (4',6-diamidino-2-phenylindole; blue), respectively. (b,d,f) The same sections stained for Mcm2 (green). Images were captured using a × 40 objective. (g) Per cent of Mcm2+ cells that were also positive for IdU incorporation in SVZ sections from R26-M2rtTA;TRE-Tight-Cdkn1b mice untreated (n=4) or treated with 1 mg ml−1Dox for 3 days (n=6), 2 weeks (n=5), 5 months (n=7), or 5 months followed by removal from Dox for 1 day (5 Months 1dR,n=6). Error bars indicate s.d. IdU incorporation is reduced in treated relative to control mice (3 days,ρ=0.00014; 2 weeks,ρ=0.00017; 5 monthsρ=0.00017; two-tailed Student’st-tests) but returns to levels that are not significantly different from control on Dox removal (ρ=0.067; two-tailed Student’st-tests). (h) Clonogenic neurosphere assays where the per cent of wells in 96-well plates (n=4, error bars indicate s.d.), cultured in the absence of Dox, which contained neurospheres after one or three passages is shown for R26-M2rtTA control (blue bars) and R26-M2rtTA;TRE-Tight-Cdkn1b (red bars) mice that had been continuously treated with 1 mg ml−1Dox from 2 months through 16 months of age. More neurospheres are recovered from Cdkn1b-overexpressing mice than controls (passage 1,ρ=0.032; passage 3,ρ=0.013; two-tailed Student’st-tests). (c–l) Muscle fibres from the gastrocnemius muscles of R26-M2rtTA control (i,k) and R26-M2rtTA;TRE-Tight-Cdkn1b (j,l) mice treated with 0.25 mg ml−1Dox from months 2 to 7, and IdU during the final 3 weeks. (i,j) Pax7 (red) and DAPI (blue) overlain on a bright-field image (arrows, Pax7+ nuclei). (k,l) IdU (red) and DAPI (blue; arrows, IdU-positive nuclei). (n) Total, Pax7-negative and Pax7-positive nuclei per myofibre, and (m) per cent of nuclei labelled with IdU (n) were quantified. Scale bars ina–fandi–lindicate 50 μm. Figure 3: Proliferating and replication competent cells in the brain and muscles of R26-M2rtTA;TRE-Tight-Cdkn1b mice. Supraventricular zones from R26-M2rtTA;TRE-Tight-Cdkn1b mice either untreated ( a , b ) or treated with 1 mg ml −1 doxycycline (Dox) between months 2 and 7 ( c , d ) or treated between months 2 and 7 but removed from Dox treatment for 24 h ( e , f ). IdU was administered for 3 days ( a – d ) or 1 day ( e , f ) and CldU was administered 2 h before killing. ( a , c , e ) Stained for IdU (red), CldU (green) and DAPI (4',6-diamidino-2-phenylindole; blue), respectively. ( b , d , f ) The same sections stained for Mcm2 (green). Images were captured using a × 40 objective. ( g ) Per cent of Mcm2+ cells that were also positive for IdU incorporation in SVZ sections from R26-M2rtTA;TRE-Tight-Cdkn1b mice untreated ( n =4) or treated with 1 mg ml −1 Dox for 3 days ( n =6), 2 weeks ( n =5), 5 months ( n =7), or 5 months followed by removal from Dox for 1 day (5 Months 1dR, n =6). Error bars indicate s.d. IdU incorporation is reduced in treated relative to control mice (3 days, ρ =0.00014; 2 weeks, ρ =0.00017; 5 months ρ =0.00017; two-tailed Student’s t -tests) but returns to levels that are not significantly different from control on Dox removal ( ρ =0.067; two-tailed Student’s t -tests). ( h ) Clonogenic neurosphere assays where the per cent of wells in 96-well plates ( n =4, error bars indicate s.d. ), cultured in the absence of Dox, which contained neurospheres after one or three passages is shown for R26-M2rtTA control (blue bars) and R26-M2rtTA;TRE-Tight-Cdkn1b (red bars) mice that had been continuously treated with 1 mg ml −1 Dox from 2 months through 16 months of age. More neurospheres are recovered from Cdkn1b-overexpressing mice than controls (passage 1, ρ =0.032; passage 3, ρ =0.013; two-tailed Student’s t -tests). ( c – l ) Muscle fibres from the gastrocnemius muscles of R26-M2rtTA control ( i , k ) and R26-M2rtTA;TRE-Tight-Cdkn1b ( j , l ) mice treated with 0.25 mg ml −1 Dox from months 2 to 7, and IdU during the final 3 weeks. ( i , j ) Pax7 (red) and DAPI (blue) overlain on a bright-field image (arrows, Pax7+ nuclei). ( k , l ) IdU (red) and DAPI (blue; arrows, IdU-positive nuclei). ( n ) Total, Pax7-negative and Pax7-positive nuclei per myofibre, and ( m ) per cent of nuclei labelled with IdU ( n ) were quantified. Scale bars in a – f and i – l indicate 50 μm. Full size image To determine whether the reduction in cell division evidenced by reduced nucleoside analogue incorporation resulted from loss of stem and progenitor cells, the presence of Mcm2-expressing cells (Mcm2 marks cells, which are competent for replication [23] ) was compared for control and 1 mg ml −1 doxycycline-treated R26-M2rtTA;TRE-Tight-Cdkn1b mice ( Fig. 3b,d and Supplementary Fig. S1 ). These studies demonstrate that despite reduced proliferation, Mcm2-expressing cells remain present in the SVZ during prolonged doxycycline treatment at levels that are similar to those found in untreated control animals. To confirm that these cells remain capable of entering the cell cycle, R26-M2rtTA;TRE-Tight-Cdkn1b mice that had been administered 1 mg ml −1 doxycycline continuously for 5 months were removed from doxycycline treatment for a period of 24 h and simultaneously labelled with IdU. Mice were additionally labelled with CldU during the final 2 h after doxycycline removal ( Fig. 3e,f ). These studies demonstrate that Mcm2-expressing cells resume cycling within 24 h after doxycycline removal, to nearly the level observed in untreated control animals ( Fig. 3g ). To confirm that stem cell levels in the brain are unaffected by prolonged Cdkn1b overexpression, neurosphere cultures were prepared in microtitre wells at limiting dilution from control ((R26-M2rtTA+ littermates that do not carry TRE-Tight-Cdkn1b) and R26-M2rtTA;TRE-Tight-Cdkn1b mice after continuous treatment with 1.0 mg ml −1 doxycycline for a period of 14 months. Cultures were maintained in the absence of doxycycline and the numbers of neurospheres present after 10 days of culture, or after two re-passages, were determined ( Fig. 3h ). For both the initial cultures and following re-passaging, the number of neurospheres recovered from mice that had been continuously treated with doxycycline for over 1 year was similar to or higher than that for controls. Together, these results show that although the rate of proliferation of neural stem/progenitor cells in Cdkn1b-overexpressing mice is reduced, these cells remain present at levels similar to control animals. The frequency of muscle stem and progenitor cells was also assessed for the gastrocnemius muscle in R26-M2rtTA;TRE-Tight-Cdkn1b transgenic mice treated (beginning at 2 months of age) with 0.25 mg ml −1 doxycycline for 5 months and controls (R26-M2rtTA+ littermates that do not carry TRE-Tight-Cdkn1b but were treated with doxycycline in parallel) using Pax7 as a stem/progenitor cell marker [24] (Fig. 3i,j ). The number of Pax7-positive and -negative nuclei per muscle fibre were determined ( Fig. 3m ). The total number of nuclei associated with the sections of each fibre is modestly reduced in Cdkn1b-overexpressing mice, from 1.9 to 1.6. A larger shift occurs in the distribution between Pax7-negative and -positive nuclei, where the frequency of Pax7-negative nuclei is reduced by over 1/3, from 1.7 to 1.0 nuclei per fibre, whereas the frequency of Pax7-positive nuclei per fibre is nearly tripled, shifting from ~0.2 in control animals to ~0.6 in Cdkn1b-overexpressing mice. As, in wt mice, Pax7 is known to be expressed in satellite cells and rapidly proliferating, transient amplifying progeny, one explanation for this shift is that delayed replication in the transient amplifying population results in cells stalling at this step of differentiation with a resulting reduction in contribution to muscle fibres. Consistent with this observation, long-term labelling of muscle with IdU (3 weeks) demonstrated that the number of nuclei incorporating IdU decreased to ~20% of the wt levels in Cdkn1b-overexpressing mice ( Fig. 3k,l,n ). The effect of Cdkn1b overexpression on cell proliferation in the small intestine was also examined. R26-M2rtTA;TRE-Tight-Cdkn1b transgenic mice were treated with doxycycline for various periods and administered IdU (3 days) and CldU (2 h) before killing. The number of crypt nuclei incorporating CldU during a 2-h labelling period is reduced to ~2% of wt values at 3 days of doxycycline administration in R26-M2rtTA;TRE-Tight-Cdkn1b mice (from 23.1 (s.d., 3.3) to 0.45 (s.d., 0.6); Fig. 4a versus Fig. 4b , green). In these animals, no crypts were observed to contain more than three labelled nuclei, and over 60% of the crypts contained no labelled nuclei. In addition, all crypts exhibit evidence of Cdkn1b overexpression ( Fig. 4b , red). Nonetheless, IdU administration over a 3-day period resulted in a high proportion of labelled cells, demonstrating that the effect of Cdkn1b overexpression is to slow, rather than block, cell cycling ( Fig. 4e , red). 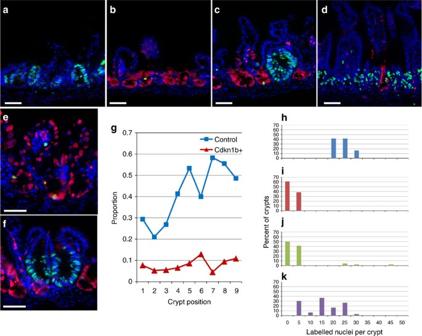Figure 4: CldU incorporation and Cdkn1b expression in the ileums of doxycycline (Dox)-treated R26-M2rtTA;TRE-Tight-Cdkn1b mice. M2rtTA; TRE-Tight-Cdkn1b mice were either untreated (a) or treated continuously at 2 months of age with 1 mg ml−1Dox for 3 days (b,e), 2 weeks (c,f) or 5 months (d). Paraffin sections were prepared and stained for CldU incorporation (green) and Cdkn1b (red) (a–d,f), or CldU (green) and IdU (red) incorporation (e), and images were captured using a × 20 objective. Ing, the frequency with which Mcm2+ nuclei (seeSupplementary Fig. S2) at various positions from the bases of the crypts label with CldU after a 2-h pulse is quantified for control (blue squares) and Cdkn1b-overexpressing (red triangles) mice. Inh–k, the distribution of crypts containing different numbers of nuclei incorporating CldU is plotted for untreated (h) and 3 days (i), 2 week (j) and 5 month (k) Dox-treated mice. Scale bars ina–findicate 50 μm. Figure 4: CldU incorporation and Cdkn1b expression in the ileums of doxycycline (Dox)-treated R26-M2rtTA;TRE-Tight-Cdkn1b mice. M2rtTA; TRE-Tight-Cdkn1b mice were either untreated ( a ) or treated continuously at 2 months of age with 1 mg ml −1 Dox for 3 days ( b , e ), 2 weeks ( c , f ) or 5 months ( d ). Paraffin sections were prepared and stained for CldU incorporation (green) and Cdkn1b (red) ( a – d , f) , or CldU (green) and IdU (red) incorporation ( e ), and images were captured using a × 20 objective. In g , the frequency with which Mcm2+ nuclei (see Supplementary Fig. S2 ) at various positions from the bases of the crypts label with CldU after a 2-h pulse is quantified for control (blue squares) and Cdkn1b-overexpressing (red triangles) mice. In h – k , the distribution of crypts containing different numbers of nuclei incorporating CldU is plotted for untreated ( h ) and 3 days ( i ), 2 week ( j ) and 5 month ( k ) Dox-treated mice. Scale bars in a – f indicate 50 μm. Full size image Prior studies have shown that the base of the small intestinal crypt contains two types of cells, that is, crypt basal columnar (CBC) cells (all of which express the wnt-responsive G protein-coupled receptor Lgr5 (ref. 25 ) and Paneth cells. CBC cells have been shown to be the predominant active stem cells within the small intestine, and clonal tracing data supports that these cells undergo frequent symmetric divisions to give rise to either two transient amplifying cells, which move up the crypt and, after several rapid divisions, differentiate to epithelial lineages, or two basal columnar cells that replace stem cells lost to differentiation [26] . The replication licensing factor Mcm2 is expressed in all CBC cells and transit amplifying cells, but not in Paneth cells [27] ( Supplementary Fig. S2a ). Measurement of the proportion of Mcm2+ cells incorporating CldU at different positions within Cdkn1b-overexpressing crypts of 3 days and 2 weeks doxycycline-treated mice demonstrates that proliferation is reduced in both CBC stem cells at the crypt base and progenitor cells at higher positions within the crypts ( Fig. 4g ). This observation demonstrates that Cdkn1b overexpression suppresses cell division in both stem and transit amplifying cells. In addition, these studies show that similar to that for transit amplifying cells, the number of Mcm2+ CBC stem cells is progressively reduced during Cdkn1b overexpression ( Supplementary Fig. S2B–J ). Depletion of stem cells is not expected if these cells undergo invariant asymmetric division but is consistent with a symmetric, neutral drift model of stem cell division [26] . Following longer periods of doxycycline treatment, CldU labelling demonstrates that a subset of crypts exhibit more active cell cycling. At 2 weeks of doxycycline treatment ( Fig. 4b ), ~8% of the crypts contain as many or more labelled nuclei than crypts of control animals ( Fig. 4c,f,i ). These crypts exhibit morphology consistent with crypts undergoing fission ( Fig. 4c,f ; green). In addition, crypts containing rapidly cycling cells fail to exhibit Cdkn1b overexpression ( Fig. 4c,f ; red). After 5 months of continuous doxycycline treatment, most crypts contain a high proportion of CldU-labelled cells, similar to controls, and fail to exhibit Cdkn1b overexpression, although evidence of Cdkn1b overexpression and a reduced rate of cycling are still found in ~1/4 of the crypts ( Fig. 4d,j ). These results are consistent with prior studies demonstrating that the intestine has an exceptional ability to eliminate stem cells that divide at suboptimal rates [27] , [28] , [29] , [30] , [31] , [32] . It is likely to be that survival of Cdkn1b-overexpressing mice depends on replacement of the majority of the intestinal epithelia with cells in which the transgene is no longer expressed and that the early loss of a fraction of Cdkn1b-overexpressing mice, particularly at the highest doses of doxycycline, results from insufficient intestinal function. DNA damage response and cellular senescence To address the possibility that Cdkn1b overexpression caused tissue degeneration through increased genetic damage and induction of a DNA damage response, ser18 phosphorylation of p53, a key event in the DNA damage response was measured. The levels of pp53 (ser18) were determined in several tissues of 4-month-old Cdkn1b-overexpressing mice and compared with levels in 4- and 24-month-old controls ( Fig. 5a ). Rather than showing elevated levels, as might be expected if Cdkn1b expression results in increased genetic damage, pp53 (ser18) levels are reduced in many different tissues of Cdkn1b-overexpressing mice. Consistent with reduced pp53 (ser18) levels, the frequency of cells with γ-H2AX and TP53bp1 foci is reduced in the epidermis of Cdkn1b-overexpressing mice ( Fig. 5b–g ; similar results were obtained for γ-H2AX foci in SVZ cells, Supplementary Fig. S3 ). The possibility that elevated Cdkn1b levels induce cellular senescence was assessed by measuring the level of senescence-associated β-galactosidase (SAβgal) activity in abdominal fat, a tissue in which SAβgal activity is known to increase during ageing, and in progeroid mouse models of ageing [5] . Even though the total abdominal fat is reduced in Cdkn1b-overexpressing mice, the SAβgal activity is not elevated in this tissue relative to controls ( Fig. 5h ). Interleukin-6, a prominent cytokine expressed in DNA damage-induced senescent cells [33] , is also not elevated in Cdkn1b-overexpressing mice ( Supplementary Fig. S4 ), consistent with the lack of accumulation of senescent cells. Finally, prior studies of Skp2-null mice, in which Cdkn1b is overexpressed to levels similar to those achieved here, have shown that nuclear enlargement and polyploidy occur within a subset of tissues, including the tubular epithelia of the kidney [21] . However, Skp2-null mice also overexpress cyclin E (ref. 21 ), and polyploidy within these tissues may result from cyclin E, rather than Cdkn1b, overexpression. Nuclear enlargement is not observed in the kidney tubular epithelial cells in Cdkn1b-overexpressing mice ( Supplementary Fig. S5 ), demonstrating that Cdkn1b overexpression alone is not responsible for this phenotype of Skp2-null mice. 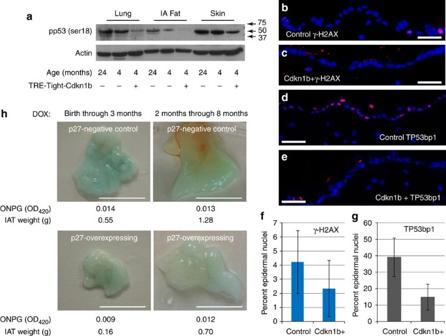Figure 5 (a) Western blottings for pp53 (ser18) (a full-length image of this blot is shown inSupplementary Fig. 10b) and actin in the lung, intra-abdominal fat (IA fat) and skin of R26-M2rtTA transgenic mice that either carry or do not carry the TRE-Tight-Cdkn1b transgene as indicated in the figure, where, starting at 2 months of age, mice were continuously treated with 1 mg ml−1doxycycline (Dox) for 2 months and assessed at 4 months of age. In addition, Cdkn1b expression in the same tissues from a control 24-month-old mouse is included for comparison. Arrows indicate the positions of size markers in kDa. (b,c) Immune-fluorescence staining for γ-H2AX in epidermal sections of control (b) and Cdkn1b-overexpressing (c) mice. (d,e) Immune-fluorescence staining for TP53BP1 in epidermal sections of control (d) and Cdkn1b-overexpressing (e) mice. (f,g) reduced frequency of γ-H2AX (n=9, error bars indicate s.d.,ρ=0.04, two-tailed Student’st-test) and TP53BP1 (n=10, error bars indicate s.d,ρ=3.7 × 10−5, two-tailed Student’st-test) foci, respectively, in epidermal sections from Cdkn1b-overexpressing mice relative to controls. (h) SAβgal staining of intra-abdominal fat (IAT) for R26-M2rtTA control and R26-M2rtTA;TRE-Tight-Cdkn1b transgenic mice that were treated with 1 mg ml−1Dox either from birth through 3 months of age (left panels) or starting at 2 months of age and through 8 months of age (right panels). Scale bar, 5 mm. Quantitative assessment of SAβgal activity was made using ONPG (O-nitrophenyl-β-galactoside) as a substrate and results from this assay are shown below each panel. In addition, the weight of total IAT recovered from each animal is given in grams. Qualitatively similar SAβgal staining was observed in two additional sets of control and R26-M2rtTA;TRE-Tight-Cdkn1b mice treated with 0.25 mg ml−1Dox from months 2 to 7, although quantitative measures were not performed. Figure 5 (a) Western blottings for pp53 (ser18) (a full-length image of this blot is shown in Supplementary Fig. 10b ) and actin in the lung, intra-abdominal fat (IA fat) and skin of R26-M2rtTA transgenic mice that either carry or do not carry the TRE-Tight-Cdkn1b transgene as indicated in the figure, where, starting at 2 months of age, mice were continuously treated with 1 mg ml −1 doxycycline (Dox) for 2 months and assessed at 4 months of age. In addition, Cdkn1b expression in the same tissues from a control 24-month-old mouse is included for comparison. Arrows indicate the positions of size markers in kDa. ( b , c ) Immune-fluorescence staining for γ-H2AX in epidermal sections of control ( b ) and Cdkn1b-overexpressing ( c ) mice. ( d , e ) Immune-fluorescence staining for TP53BP1 in epidermal sections of control ( d ) and Cdkn1b-overexpressing ( e ) mice. ( f , g ) reduced frequency of γ-H2AX ( n =9, error bars indicate s.d., ρ =0.04, two-tailed Student’s t -test) and TP53BP1 ( n =10, error bars indicate s.d, ρ =3.7 × 10 −5 , two-tailed Student’s t -test) foci, respectively, in epidermal sections from Cdkn1b-overexpressing mice relative to controls. ( h ) SAβgal staining of intra-abdominal fat (IAT) for R26-M2rtTA control and R26-M2rtTA;TRE-Tight-Cdkn1b transgenic mice that were treated with 1 mg ml −1 Dox either from birth through 3 months of age (left panels) or starting at 2 months of age and through 8 months of age (right panels). Scale bar, 5 mm. Quantitative assessment of SAβgal activity was made using ONPG ( O -nitrophenyl-β-galactoside) as a substrate and results from this assay are shown below each panel. In addition, the weight of total IAT recovered from each animal is given in grams. Qualitatively similar SAβgal staining was observed in two additional sets of control and R26-M2rtTA;TRE-Tight-Cdkn1b mice treated with 0.25 mg ml −1 Dox from months 2 to 7, although quantitative measures were not performed. Full size image Reversibility of the Cdkn1b-overexpressing phenotype The observations above demonstrate that despite degenerative changes, adult mice overexpressing Cdkn1b for long periods of time retain neural stem/progenitor and muscle satellite cells. The continued presence of these cells and the lack of evidence for accumulation of senescent cells raise the possibility that many of the phenotypic changes resulting from Cdkn1b overexpression might be reversed on return of Cdkn1b to wt levels after the removal of doxycycline. To test this possibility, R26-M2rtTA;TRE-Tight-Cdkn1b mice that had been continuously treated with doxycycline for 8 or more months were removed from doxycycline treatment and were monitored for reversal of phenotypic changes. Surprisingly, these mice showed little improvement at a gross phenotypic level, and some aspects of their condition declined more rapidly when removed from doxycycline treatment than observed for mice that were continued on doxycycline for similar or longer periods ( Fig. 6a ). In particular, the removal of Cdkn1b-overexpressing mice from doxycycline treatment resulted in exacerbation of skin lesions that limited the time over which the mice could be followed. 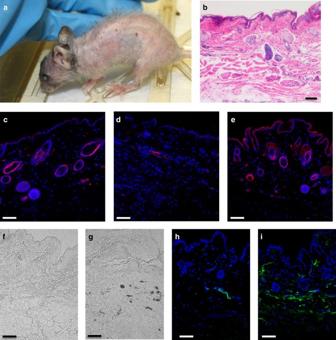Figure 6: Effect of doxycycline (Dox) removal on the gross phenotype and skin of R26-M2rtTA;TRE-Tight-Cdkn1b mice. The phenotype of an R26-M2rtTA;TRE-Tight-Cdkn1b mouse treated with 0.75 mg ml−1Dox from 2 through 9 months of age followed by removal from doxycycline for three additional months is shown ina(where the same animal is shown before removal from Dox treatment inFig. 1g). (b–i) Images of histological sections from the abdominal skin of this mouse wherebis haematoxylin and eosin stained and taken with a × 10 objective; (d–e) Immuno-fluorescence images stained for smooth muscle actin (red) and DAPI (4',6-diamidino-2-phenylindole; blue), and taken with a × 20 objective. (f,g) Unstained phase-contrast images taken with a × 20 objective. (h,i) Immuno-fluorescence images stained for IgG (green) and DAPI (blue), and taken with a × 20 objective. (c,f,h) Controls prepared from an R26-M2rtTA mouse treated with Dox; (d) from an R26-M2rtTA;TRE-Tight-Cdkn1b mouse treated continuously with Dox; and (e,g,i) from an R26-M2rtTA;TRE-Tight-Cdkn1b mouse following treatment with and removal from Dox as described above. Scale bars inb–iindicate 50 μm. Figure 6: Effect of doxycycline (Dox) removal on the gross phenotype and skin of R26-M2rtTA;TRE-Tight-Cdkn1b mice. The phenotype of an R26-M2rtTA;TRE-Tight-Cdkn1b mouse treated with 0.75 mg ml −1 Dox from 2 through 9 months of age followed by removal from doxycycline for three additional months is shown in a (where the same animal is shown before removal from Dox treatment in Fig. 1g ). ( b – i ) Images of histological sections from the abdominal skin of this mouse where b is haematoxylin and eosin stained and taken with a × 10 objective; ( d – e ) Immuno-fluorescence images stained for smooth muscle actin (red) and DAPI (4',6-diamidino-2-phenylindole; blue), and taken with a × 20 objective. ( f , g ) Unstained phase-contrast images taken with a × 20 objective. ( h , i ) Immuno-fluorescence images stained for IgG (green) and DAPI (blue), and taken with a × 20 objective. ( c , f , h ) Controls prepared from an R26-M2rtTA mouse treated with Dox; ( d ) from an R26-M2rtTA;TRE-Tight-Cdkn1b mouse treated continuously with Dox; and ( e , g , i ) from an R26-M2rtTA;TRE-Tight-Cdkn1b mouse following treatment with and removal from Dox as described above. Scale bars in b – i indicate 50 μm. Full size image Histological sections of the skin from 12-month-old control (R26-M2rtTA+ mice that do not carry TRE-Tight-Cdkn1b but which were treated with doxycycline) and R26-M2rtTA;TRE-Tight-Cdkn1b mice continuously treated with doxycycline for 9 months and removed from doxycycline treatment for 3 months are shown in Fig. 6b–i . Thinning of the hypodermal layer is not reversed in mice removed from doxycycline treatment ( Fig. 6b ). Nonetheless, cell density within dermal and epidermal layers is increased. Hair follicles and sebaceous glands are more prominent in the dermal layer, and many of the new cells stain for smooth muscle actin expression in both the epidermal and dermal layers ( Fig. 6c–e ). Unstained phase-contrast images are shown in Fig. 6f,g and demonstrate the presence of pockets of melanocytes in mice removed from doxycycline treatment (brown spots are also observed in the skin of live mice, Fig. 6a ). Deposition of IgG is also observed ( Fig. 6h,i ). The effect of Cdkn1b overexpression on CD34+ putative stem cells within the hair follicle bulge was also assessed ( Supplementary Fig. S6 ). CD34+ cells are reduced to ~1/4 of control numbers in mice continuously overexpressing Cdkn1b; however, within the hair follicles that remain, the frequency of these cells recovers to near-control levels in mice that have been removed from doxycycline treatment. The effect of doxycycline removal on the ratio of lymphoid to myeloid cells within the peripheral blood was also determined. Mice treated continuously with doxycycline show a reduction in this ratio from ~8.4 to ~2.1 ( Supplementary Fig. S7a,b ). Removal of doxycycline does not result in a reversal of the effect through at least 7 weeks ( Supplementary Fig. S7c ). Despite failure to reverse lymphoid/myeloid ratios in the blood and the worsened condition of the skin, there is evidence of recovery in some tissues of Cdkn1b mice after the removal from doxycycline treatment. Both the gastrocnemius and abdominal muscles show substantial recovery of muscle fibre diameter following doxycycline removal ( Supplementary Fig. S8 ). There is, in addition, an increase in nuclei associated with each muscle fibre. However, these improvements are accompanied by an increased infiltration of adipose tissue. The infiltration of the muscle with adipose tissue and an increased presence of melanocyctes and myofibroblasts within the skin are changes that frequently accompany normal ageing of these tissues. Although such changes may occur in response to tissue degeneration in normally ageing tissues, they may be suppressed by reduced proliferation in animals continuously overexpressing Cdkn1b. Overgrowth of subsets of cells on release from this proliferation block could account for the more rapid decline of Cdkn1b-overexpressing mice that have been removed from doxycycline treatment relative to those that are continued on doxycycline treatment. These observations suggest that loss of tissue organization and irreversibility of compensatory changes may contribute significantly to the degeneration of some tissues during ageing. Cdkn1b overexpression in neonatal mice Prior studies have shown that Cdkn1b is overexpressed throughout the development process in most tissues of Skp2-null mice [21] . Although these mice are smaller, they do not exhibit progeroid phenotypes. To examine the effect of Cdkn1b overexpression on immature mice, nursing mothers with newborn litters of neonatal R26-M2rtTA mice, either carrying or not carrying the TRE-Tight-Cdkn1b transgene, were treated with 1 mg ml −1 doxycycline, and weights of the animals were determined weekly, beginning at 3 weeks and through 15 weeks of age ( Fig. 7a ). Cdkn1b-overexpressing mice show a reduced rate of growth during the period between 4 and 10 weeks of age, during which non-transgenic animals grow nearly exponentially to more than double in weight. In contrast, Cdkn1b-overexpressing animals exhibit a more linear weight gain such that the greatest differences between control and Cdkn1b-overexpressing mice occur between weeks 4 and 6, during which the weight of control animals is nearly double that of the Cdkn1b-overexpressing animals. Morphologically, Cdkn1b-overexpressing mice exhibit an obvious developmental delay during this period ( Fig. 7b,d,e ). Despite the developmental delay, mice in which Cdkn1b is overexpressed during neonatal development show a significant reduction in degenerative phenotypes relative to mice that were initially treated with doxycycline for similar durations but beginning at 2-months of age (compare Fig. 7d–g with Fig. 7h–k ). The improved phenotypes include reduced loss of hair and pigmentation, thicker skin with fewer lesions and greater corneal transparency. Improvements are also apparent in histological sections of the skin and muscle relative to age-matched controls ( Supplementary Fig. S9 ). Tissue sections from control and Cdkn1b-overexpressing mice are shown for the gastrocnemius muscle in panels a and b, and the abdominal muscles in panels c and d. Fibre diameters were determined (panel e) and demonstrate no significant difference between control and Cdkn1b-overexpressing mice for either of these muscles. Skin thickness is also similar between the 8-week-old control and Cdkn1b-overexpressing mice, (Supplementary Figs S9f,g). Nonetheless, the number of cells incorporating the nucleoside analogue is reduced ( Supplementary Fig. S9h–j ) consistent with the delayed growth of these animals. R26-M2rtTA;TRE-Tight-Cdkn1b transgenic mice treated with doxycycline as neonates eventually achieve body mass similar to that of controls at which point the degenerative phenotypes become apparent ( Fig. 7c ). These results are consistent with the idea that a key determinate of whether degenerative phenotypes are observed at the tissue level is the ratio between cell proliferation and the mass of the tissue that must be maintained. 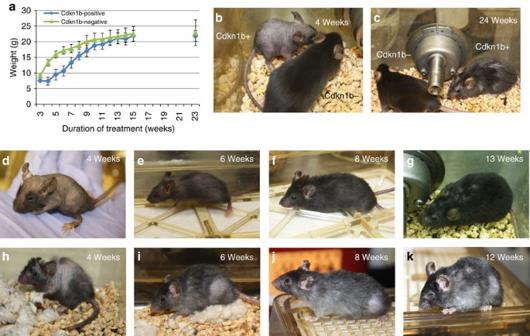Figure 7: Phenotypic effects of Cdkn1b overexpression in neonatal versus adult animals. (a) Weight in grams of R26-M2rtTA;TRE-Tight-Cdkn1b (n=22) and R26-M2rtTA control (n=21) littermates during neonatal development when mothers were treated with 0.25 mg ml−1doxycycline (Dox) on birth of the pups (error bars indicate s.d.). (b) Comparison of an R26-M2rtTA;TRE-Tight-Cdkn1b (Cdkn1b+) with an R26-M2rtTA (Cdkn1b−) control littermate at 4 weeks of development after continuous treatment with 0.25 mg ml−1Dox. (c) The same pair of animals after 24 weeks of continuous Dox administration. (d–k) Comparison of mice treated for various times with 0.25 mg ml−1Dox either as neonates (d–g) or when treatment was begun at 2 months of age (h–k), (d,h) 4 weeks of treatment, (e,i)6 weeks of treatment, (f,j) 8 weeks of treatment and (g,k) 12–13 weeks of treatment. Figure 7: Phenotypic effects of Cdkn1b overexpression in neonatal versus adult animals. ( a ) Weight in grams of R26-M2rtTA;TRE-Tight-Cdkn1b ( n =22) and R26-M2rtTA control ( n =21) littermates during neonatal development when mothers were treated with 0.25 mg ml −1 doxycycline (Dox) on birth of the pups (error bars indicate s.d.). ( b ) Comparison of an R26-M2rtTA;TRE-Tight-Cdkn1b (Cdkn1b+) with an R26-M2rtTA (Cdkn1b−) control littermate at 4 weeks of development after continuous treatment with 0.25 mg ml −1 Dox. ( c ) The same pair of animals after 24 weeks of continuous Dox administration. ( d – k ) Comparison of mice treated for various times with 0.25 mg ml −1 Dox either as neonates ( d – g ) or when treatment was begun at 2 months of age ( h – k ), ( d , h ) 4 weeks of treatment, ( e , i) 6 weeks of treatment, ( f , j ) 8 weeks of treatment and ( g , k ) 12–13 weeks of treatment. Full size image Cdkn1b is a key regulator of cell cycle progression that was initially identified based on its induction by extracellular antiproliferative signals, including contact inhibition or serum deprivation. Similar to other members of this family, Cdkn1a (p21) and Cdkn1c (p57), Cdkn1b has the ability to bind to the cyclin-cyclin dependent kinase (CDK) holoenzyme and inhibit CDK complexes required for G1 progression and S-phase entry. It is known to inhibit cell cycle progression when overexpressed in essentially all cell types in culture. Consistent with results from cultured cells, adult mice in which overexpression of Cdkn1b is broadly induced demonstrate reduced levels of cell proliferation in all of the tissues examined (SVZ, skeletal muscle, skin and transiently in the intestine) in the present study. Many of the degenerative changes observed in Cdkn1b-overexpressing mice are likely to be a consequence of reduced cell proliferation. Additional functions for Cdkn1b have been described. Cytoplasmic Cdkn1b has been shown to regulate the actin cytoskeleton and affect cell migration by modulation of Rho [34] . This function of Cdkn1b could contribute to some of the phenotypes observed in the present study (for example, failure of SVZ progenitors to migrate to the olfactory bulb or failure of muscle satellite cells to fuse to myofibrils). Cdkn1b has also been shown to interact in a transcriptional repressor complex [35] and loss of Cdkn1b results in elevated Sox2 expression in multiple tissues, including the fibroblasts, lung, retina and brain [36] . Sox2 is known to be expressed in and contribute to the stem cell phenotype of a number of somatic stem cells [37] , [38] , [39] and reduced Sox2 expression could result in loss of adult stem cells. However, it is unclear that wt levels of Cdkn1b are limiting for Sox2 repression and elevating Cdkn1b levels over wt may not result in a further reduction. The increase in SVZ and muscle stem and progenitor cells is also not consistent with this role. The number of CBC stem cells per crypt is reduced in the small intestine following inhibition of cell division by Cdkn1b overexpression. Although it is possible that this loss is a direct result of a transcriptional repressor function of Cdkn1b, the mode of stem cell division in this tissue could also explain the observation. Prior studies have shown that intestinal crypt homeostasis is maintained by competition between symmetrically dividing stem cells [26] such that over time the individual stem cell lineages become fixed or extinct. Cdkn1b reduces the rate of division of CBC stem cells and, unlike the case for an invariant asymmetric mode of division, reduced division of the stem cell pool is expected to result in the observed reduction of these cells. A smaller pool of stem cells is expected to increase the rate at which individual stem cell lineages become fixed or undergo extinction within a crypt. Further, the likelihood that all stem cells within a crypt are lost to differentiation is increased and would result in a reduction in the number of intestinal crypts were it not for replacement by crypt fission. A reduced rate of cell proliferation of stem cell within hair follicles may also account for the effects of Cdkn1b overexpression within this tissue. Similar to the intestine, the number of Cd34+ stem cells present in the bulge of each follicle decreases when cell proliferation is suppressed by Cdkn1b overexpression. Loss of hair follicles due to a complete loss of stem cells within a follicle could account for alopecia in these mice. On removal of doxycycline, a number of Cd34+ stem cells recovers in the remaining follicles; however, very little reversal of alopecia is observed, consistent with a lack of generation of new follicles by fission. Additional studies will be necessary to determine whether the mode of division of lymphoid or myeloid-biased haematopoietic stem cells and the architecture of the haematopoietic stem cell niche have a role in the lymphoid-to-myeloid shift resulting from Cdkn1b overexpression or the failure to recover wt ratios after doxycycline removal. A variety of mouse models in which genome stability is compromised have been shown to exhibit a progeroid phenotype where the phenotype is thought to result from activation of the DNA damage response and the accumulation of senescent cells. For example, loss of telomerase results in an impaired tissue maintenance and a shortened life span, where these consequences are thought to result from elevated genetic damage caused by telomere dysfunction [40] . However, the effect of genetic damage on the ageing phenotype may be indirect and result from reduced cell proliferation and induction of a senescent phenotype mediated by the DNA damage response. Consistent with this idea, Cdkn1a (p21) deletion improves stem cell function and partially rescues the life span of mice with dysfunctional telomeres [9] . Further, progeroid mice in which Trp53 is constitutively hyperactive (p53+/m) exhibit reduced cell cycling, which may be a consequence of an elevated DNA damage response to normal rates of genetic damage [41] , [42] . The number of senescent cells is also increased in tissues of p53+/m mice compared with that of wt mice [42] . BubR1 is a key inhibitor of the E3 ubiquitin ligase APC/CCdc20, which, among other functions, regulates chromosome segregation. BubR1 hypomorphic mice exhibit elevated levels of aneuploidy and, in a variety of tissues, degeneration at early ages [5] . Conversely, strengthening the mitotic checkpoint through elevated levels of BubR1 has been shown to reduce genetic damage accumulation and to extend the healthy life span of mice [43] . Within a subset of tissues of BubR1 hypomorphic mice (including the skeletal muscle fat and eye), p16 Ink4a is expressed at chronically high levels, presumably in response to DNA damage. These tissues exhibit elevated levels of SAβgal and other markers of senescence and reduced levels bromodeoxyuridine (BrdU)-incorporating cells. Further, BubR1 hypomorphic mice lacking p16 Ink4a and mice in which p16 Ink4a -expressing cells are continuously ablated ameliorate degenerative changes specifically in these tissues and exhibit increased numbers of BrdU-incorporating cells [10] , [44] . It has been hypothesized that degenerative changes are a consequence of the effects of secretory changes associated with senescent cells on the tissue microenvironment [44] . The observation here that reduced cell proliferation, even in the absence of the accumulation of senescent cells, is sufficient to result in age-related degenerative changes suggests that many of the effects that senescent cells exert on the tissue microenvironment could result from suppression of cell proliferation. pp53 (Ser18) levels and DNA damage foci are reduced in proliferating tissues of Cdkn1b-overexpressing mice relative to wt animals, suggesting that replication-related errors are responsible for much of the genetic damage that occurs during ageing. Consistent with this result, cancer incidence is greatly reduced in animals in which Cdkn1b is overexpressed as adults. Further, unlike p53+/m, telomere-deficient mice or BubR1 hypomorphic mice senescent cells do not accumulate to elevated levels in Cdkn1b-overexpressing mice. Nonetheless, these mice are less robust than wt mice and exhibit degenerative tissue changes consistent with an aged phenotype. The apparent improvement in genome maintenance but reduction in tissue homeostasis suggest that Cdkn1b overexpression in adult animals alters the balance between genetic and tissue ageing. Cdkn1b expression is not increased during ageing in wt animals. Further, in skeletal muscle a subset of satellite cells has been shown to break quiescence and increase proliferation in ageing mice due to changes in growth factor signalling in the aged niche [45] . However, it is not necessary that genes contributing to an aged phenotype show a change in their level of activity during ageing, rather simply that their basal level of activity is incompatible with complete tissue maintenance over time [46] . Loss of Cdkn1b function in knockout mice results in a preferential increase in progenitor cell division relative to stem cells [47] , suggesting that endogenous Cdkn1b functions to suppress division specifically in progenitor cells but not in stem cells. Hence, the modulation of stem and progenitor cell proliferation rates achieved by overexpressing Cdkn1b in the present study is unlikely to reflect a normal role for this gene in control of stem cell division during ageing of wt mice. Nonetheless, to the extent that reduced Cdkn1b expression allows increased division of progenitors without a corresponding increase in stem cell division, the present studies suggest that partial suppression of Cdkn1b activity in ageing adult animals could improve tissue maintenance without loss of genome integrity within stem cells. Plasmid and transgenic mouse construction pTRE-Tight-Cdkn1b was constructed by insertion of a 1,261-bp fragment from pCMV-Sport6-Cdkn1b (Open Biosystems) containing the Cdkn1b coding sequence into multiple cloning site of pTRE-Tight (Invitrogen). Transgenic animals were produced by pronuclear injection of a 1.8-kbp Xho I fragment isolated from pTRE-Tight-Cdkn1b and containing the TRE promoter, Cdkn1b gene and SV40 pA into C567BL6 zygotes. One founder was identified and maintained on a C57Bl6 background using primers designed with the forward primer (TgTRE-F: 5′ GAGTTTACTCCCTATCAGTGATAGAGAACG-3′) in the TRE promoter and the reverse primer (TgTRE-R: 5′-CTCCAGGCGATCTGACGGTTC-3′) immediately downstream of the SV40 pA. The TRE-Tight-Cdkn1b mouse line is available to the research community through The Jackson Laboratory (JAX Stock Number 017631). Mouse crosses and treatments B6.Cg-Gt(ROSA)26Sor tm1(rtTA*M2)Jae /J (Jackson Laboratories, referred to as R26-M2rtTA) mice were crossed with TRE-Tight-Cdkn1b mice to generate bigenic R26-M2rtTA;TRE-Tight-Cdkn1b mice. Bigenic mice were administered doxycycline (Sigma) in their drinking water at the concentrations and durations indicated in the text. In cases where mice were labelled with IdU and CldU, IdU was administered in the drinking water at 0.5 mg ml −1 for 3 days or 3 weeks in different experiments and mice were injected with 100 μl of 10 mg ml −1 CldU in isotonic saline 2 h before the end of the experiment [23] . All procedures involving mice were approved by the Roswell Park Cancer Institute’s Institutional Animal Care and Use Committee. Immunoblotting Protein extracts from tissues were prepared using pre-chilled solutions. Tissues were collected in PBS and transferred to Eppendorf centrifuge tubes containing RIPA buffer: (20 mM Tris, pH 8.0, 150 mM NaCl, 1% NP-40 and 1% sodium deoxycholate) containing protease and phosphatase inhibitors (SigmaFast S8820 plus Phosphatase Inhibitors, Sigma; and PhosStop, catalogue number 04906845001, Roche). Tissues were homogenized in this solution and the mixture was incubated on ice for 1 h. Tubes were spun in a microcentrifuge for 40 min at 4 °C at maximum speed (14,000 r.p.m.). The supernatant was collected and protein concentrations were established by BCA assays (Thermo Scientific, catalogue number 23227). The protein concentrations were equalized between different extracts with RIPA buffer. Following immunoblotting (western blot), Cdkn1b, pp53 (ser18) and actin were detected using anti-p27(C-19; 1/1,000, catalogue number sc-528, Santa Cruz Biotechnology), anti-pp53(ser18; 1/1,000, catalogue number 9284S, Cell Signaling) or anti-actin (1/1,000, catalogue number A2066, Sigma) primary antibodies and horseradish peroxidase-conjugated anti-rabbit secondary antibody (1/2,000, AP132P GtxRb IgG (H+L) HRP, Millipore). Immunohistochemistry Tissues were paraffin embedded and 6 μm histological sections were prepared using standard techniques. Immunostaining for Cdkn1b, Pax7, myosin and Mcm2 were performed, following antigen recovery [23] , using rabbit anti-p27(C-19) (1/200, catalogue number sc-528, Santa Cruz Biotechnology), rabbit anti-Pax7 (1/200, catalogue number sc-25409, Santa Cruz Biotechnology), mouse MF20 (1/200, Developmental Studies Hybridoma Bank) and mouse BM28 (1/200, Transduction Laboratories) primary antibodies followed by Alexafluor 594-conjugated donkey anti-rabbit and Alexafluor 488-conjugated donkey anti-mouse secondary antibodies (1/500, catalogue numbers A21207 and A 20202 respectively, Invitrogen). IdU and CldU were detected for the same locations following stripping of the initial antibodies and DNA denaturation as described previously [23] Briefly, slides were treated with 1.5 m HCl for 1 h at room temperature, washed with phosphate buffered saline, treated with 0.05–0.25% trypsin for 1–15 min, depending on the tissue, and stained with mouse monoclonal anti-BrdU antibodies (1:200; cross-reactivity with IdU; Becton Dickinson, Mountain View, CA) and rat monoclonal anti-BrdU antibodies (1:200; cross-reactivity with CldU; Accurate Chemicals, Westbury, NY) at 4 °C overnight. Following wash with phosphate buffered saline, secondary anti-mouse Alexafluor 594 and anti-rat Alexafluor 486 antibodies (1:500; Santa Cruz Biotechnology) were then applied for 2 h at room temperature. Peripheral blood analysis Blood was collected from mice by retro-orbital bleeding and prepared for FACS analysis using mixture of CD4-Pacific Blue, CD8-Pacific Blue, B220-Pacific Blue, B220-PeCy7, Mac1-PeCy7 and Gr-1-PeCy7 (1/100, catalogue numbers 48-0042, 48-0081, 48-0452, 25-0452, 25-0112, and 25-5931 respectively all from eBioscience) as described previously [48] . Briefly, red blood cells were lysed and samples were incubated with antibody mixture for 20 min on ice before washing and analysis by FACS using an LSRII (Becton Dickinson). How to cite this article: Pruitt, S. C. et al. Cdkn1b overexpression in adult mice alters the balance between genome and tissue ageing. Nat. Commun. 4:2626 doi: 10.1038/ncomms3626 (2013).